Activation of the central nervous system induced by micro-magnetic stimulation Electrical and transcranial magnetic stimulations have proven to be therapeutically beneficial for patients suffering from neurological disorders. Moreover, these stimulation technologies have provided invaluable tools for investigating nervous system functions. Despite this success, these technologies have technical and practical limitations impeding the maximization of their full clinical and preclinical potential. Recently, micro-magnetic stimulation, which may offer advantages over electrical and transcranial magnetic stimulation, has proven effective in activating the neuronal circuitry of the retina in vitro . Here we demonstrate that this technology is also capable of activating neuronal circuitry on a systems level using an in vivo preparation. Specifically, the application of micro-magnetic fields to the dorsal cochlear nucleus activates inferior colliculus neurons. Additionally, we demonstrate the efficacy and characteristics of activation using different magnetic stimulation parameters. These findings provide a rationale for further exploration of micro-magnetic stimulation as a prospective tool for clinical and preclinical applications. Electrical and transcranial magnetic stimulation (TMS) of the nervous system have proven to be beneficial for patients suffering from neurological disorders including Parkinson’s disease [1] , [2] , essential tremor [3] , dystonia [4] , [5] , stroke [6] , [7] , [8] and chronic neuropathic pain [9] , [10] . These stimulation tools are also invaluable for investigating various functions of the nervous system. Despite this success, these technologies have technical and practical limitations impeding their full potential [11] , [12] . Here we investigate the use of micro-magnetic stimulation (μMS) as an alternative neuromodulatory technology, which may overcome some of the limitations of conventional electrical stimulation and TMS. Following Luigi Galvani’s discovery in the 1700s that the application of electrical current to nerves could elicit muscular contractions, electrical stimulation led to a rapid advancement in our understanding of the function and organization of the nervous system [13] . The modern use of electrical stimulation, targeting deep cerebral structures for management of neurological disorders, did not occur until the 1950s, when Robert Heath [14] implanted electrodes in patients with chronic pain. Since its reintroduction in the 1980s by Benabid et al. [15] , and termed deep brain stimulation (DBS), electrical stimulation has been used as a therapeutic modality for the treatment of a variety of neurological conditions including essential tremor, Parkinson’s disease and dystonia, and is currently being investigated for the treatment of chronic pain, major depression, obsessive-compulsive disorder and epilepsy [6] , [16] , [17] , [18] , [19] , [20] . Alternatively, according to Faraday’s law of induction, time-varying magnetic fields generated by alternating current through a coil can induce extracellular electrical fields and neuronal activation [21] . In 1896, d’Arsonval et al. [22] developed a large alternating power source that when applied to a coil external to the skull, activated neurons within the brain, providing empirical evidence to support the notion of the stimulation of nervous tissue by electromagnetic induction. However, this technology was not widely utilized until the 1980s when electronic and power source advancements led to the development of a reliable system, termed TMS [23] . In seminal studies, Barker et al. [23] were able to generate a muscle twitch response of the contralateral limbs by TMS activation of cortex. Since the development of TMS, many scientists have pioneered its use as a non-invasive means of modulating brain activity for either neuroscientific investigations or as a therapeutic modality [24] , [25] . Despite their successes, electrical and TMS therapies have efficacy, safety and practical limitations. For instance, with invasive electrical stimulation methods (such as DBS), the primary limitation is unintended oxidation and reduction at the electrode–tissue interface that can result in electrode corrosion and tissue damage [26] . Furthermore, patients with implanted neurostimulation systems live with limited access to important medical tools such as MRI and diathermy due to concerns related to device and tissue damage [27] , [28] . In contrast, non-invasive methods, such as TMS or transcranial direct current stimulation (tDCS) [29] , offer advantages over invasive neuromodulatory technologies but have limited applications. In TMS, the neuronal activation is generated via electromagnetic induction, whereas in tDCS, it is generated by electric current injection through the scalp and calvarium. In both of these methods, the brain is activated without a direct interface between neural tissue in the brain and the stimulus source. However, the application of these techniques is affected by poor reproducibility resulting from variability of induced electric field due to heterogeneous brain tissue as well as anthropomorphic factors such as shape of skull and scalp-to-cortex distance. The lack of spatial selectivity is critical because in many current and emerging applications, the target area for producing the intended effects is in the immediate vicinity of areas that, if stimulated, produce side effects [11] , [30] . In addition, TMS requires large power sources (≤20,000 A) [31] to drive the magnetic fields, as the coils are large and far from the brain tissue. Together, these limitations reduce their feasibility as chronic neurotherapeutic applications. Owing to recent advancements in micro-machining technologies, we can now utilize coils constructed on the submillimeter scale. Like the coils used in TMS, when current is applied to the microcoil, a magnetic field is generated. Temporal changes of the magnetic field induce the electrical field, which evokes action potentials. We posit that microcoils can offer advantages over classical electrical and TMS techniques. Unlike TMS coils, μMS coils are submillimeter in size and can be placed within or in close proximity to a neuronal substrate, increasing spatial resolution and reducing the power needed to evoke neuronal activity. Moreover, because the coils are not in direct contact with tissue and no current is directly injected, they may overcome safety concerns related to electrode–tissue interface. Recently μMS has proven effective in activating the local neural circuitry of the retina in vitro [32] . In this study it was demonstrated that μMS of retinal ganglion cells activates neurons, and that this activation is sensitive to the amplitude and orientation of the applied magnetic field. While this study is an important first step in demonstrating the feasibility of μMS, an important next step is to examine the effects of μMS on brain circuits in live animals and to explore how different stimulus parameters, such as amplitude and pulse-width, affect neuronal activation. Here we demonstrate that μMS is capable of activating neuronal circuitry on the systems level, using an in vivo rodent preparation to examine the cochlear nucleus (CN)–inferior colliculus (IC) auditory pathway. We chose this model because the electrophysiology and anatomy of this pathway have been well studied and characterized. Our results demonstrate that μMS of the CN trans-synaptically activates neurons in the IC. Moreover, we demonstrate the efficacy and characteristics of IC activation using different amplitudes and pulse-widths of stimulation. These findings provide a rationale for the further exploration of μMS as a prospective tool for clinical and preclinical applications. Experimental setup The trans-synaptic activation of neurons using submillimeter size coils was demonstrated by the application of μMS to the dorsal cochlear nucleus (DCN), while measuring the neuronal activity of the contralateral IC in anaesthetised hamsters ( n =6, Fig. 1 ). Specifically, microcoils ( Fig. 1b ) were oriented parallel to the medio-lateral axis of the DCN while glass pipette recording electrodes were advanced into the contralateral IC, as illustrated in Fig. 1a . Once stable auditory evoked electrophysiological signals were isolated from the IC and the threshold for neuronal activation was determined (see Methods), a computer-controlled stimulation system randomly presented different amplitudes and pulse-widths of μMS to the DCN. The different parameters of μMS were presented following a 30-s interval in which no stimulation was applied. All electrophysiology data were digitized and analysed offline. 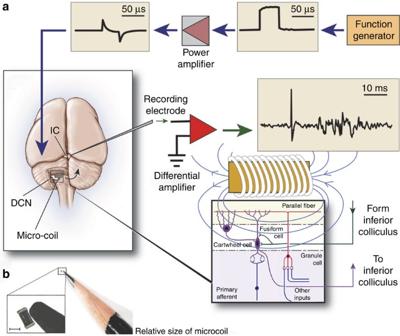Figure 1: Experimental setup and image of a microcoil. (a) Illustration of animal preparation and experimental setup. The animal was anaesthetised, and the DCN and IC were surgically exposed. Once homoeostasis was achieved, a recording electrode was placed into the IC and a microcoil was positioned over the DCN. Stimulation was then applied to the coils, using a function generator and amplifier (voltage gain: 5 × ), as electrophysiological data were simultaneously recorded from the IC. Computer control software presented different parameters of stimulation to the coils during the recording sessions. The lower right inset illustrates the positioning of the coil over the different layers of the DCN. (b) Image of a microcoil used in the study relative to a pencil point (scale bar, 500 μm). The coil used in this study is a helical square with 21 turns (400 × 400 × 600 μm, uninsulated dimension) and 100 nH inductance. Figure 1: Experimental setup and image of a microcoil. ( a ) Illustration of animal preparation and experimental setup. The animal was anaesthetised, and the DCN and IC were surgically exposed. Once homoeostasis was achieved, a recording electrode was placed into the IC and a microcoil was positioned over the DCN. Stimulation was then applied to the coils, using a function generator and amplifier (voltage gain: 5 × ), as electrophysiological data were simultaneously recorded from the IC. Computer control software presented different parameters of stimulation to the coils during the recording sessions. The lower right inset illustrates the positioning of the coil over the different layers of the DCN. ( b ) Image of a microcoil used in the study relative to a pencil point (scale bar, 500 μm). The coil used in this study is a helical square with 21 turns (400 × 400 × 600 μm, uninsulated dimension) and 100 nH inductance. Full size image Activation of the IC neurons with μMS of the DCN μMS of the DCN was capable of evoking neuronal activation of the IC in all six animals tested in the study. Although variance in the evoked response was observed between experimental animals, likely due to the relative position of the coil to the DCN in each animal, two primary responses were elicited ( Fig. 2 ). 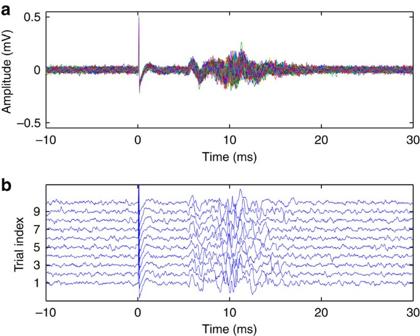Figure 2: Complex neuronal response of the IC to μMS of the DCN. (a) Illustration of overlaid electrophysiological activity from the IC in response to 100 stimulation pulses delivered to the DCN. The pulse amplitude was 500 mV, the pulse-width was 50 μs, and the average inter-pulse interval was 500 ms. As seen, the pulses generate a highly stereotypic artifact (t=0 ms), a relatively stationary consistent neuronal response (t=5–6 ms) and a longer duration non-stationary neuronal response (t=8–20 ms). (b) First 10 individual electrophysiological responses in (a). Each trace depicts the multi-unit response to individual stimulation pulses. Figure 2a illustrates overlaid electrophysiological activity from the IC in response to 100 stimulation pulses delivered to the DCN. The first response consisted of a short latency (~6 ms) synchronized neuronal activation, observed in 67% (4/6) of the animals tested. The second response consisted of a longer latency (mean latency ~15 ms), less synchronized response, observed in 100% of the animals tested. Figure 2: Complex neuronal response of the IC to μMS of the DCN. ( a ) Illustration of overlaid electrophysiological activity from the IC in response to 100 stimulation pulses delivered to the DCN. The pulse amplitude was 500 mV, the pulse-width was 50 μs, and the average inter-pulse interval was 500 ms. As seen, the pulses generate a highly stereotypic artifact ( t =0 ms), a relatively stationary consistent neuronal response ( t =5–6 ms) and a longer duration non-stationary neuronal response ( t =8–20 ms). ( b ) First 10 individual electrophysiological responses in ( a ). Each trace depicts the multi-unit response to individual stimulation pulses. Full size image The short latency-synchronized activation had little temporal variation and high reproducibility in response to each μMS pulse ( Fig. 2b ). In contrast, the long latency-evoked response was rather asynchronous and more distributed in duration, suggestive of poly-synaptic orthodromic activation [33] . Effects of μMS amplitude and pulse-width on IC activation In order to characterize the parameters of μMS, we examined the effects of different amplitudes and pulse-width of stimulation on IC activity. 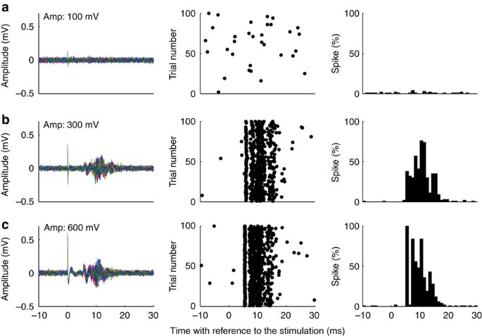Figure 3: Effects of pulse amplitude modulation on the IC neurons. Differential neuronal response of IC to low (a), intermediate (b) and high (c) amplitudes of μMS of the DCN for the same stimulation pulse-width (50 μs), while the inter-pulse interval was randomized with an average of 500 ms. The first column depicts the overlaid electrophysiological activity of the IC in response to 100 stimulation pulses delivered at each amplitude of stimulation. The second and third columns illustrate the peri-stimulus rasters and histograms of the multi-unit spiking activity, respectively. Magnetic stimulation for each plot was aligned to time equals zero. Figure 3 illustrates the effects of three different stimulus amplitudes on neuronal activity in the IC with the same pulse-width (50 μs). As shown, the lowest level of stimulation did not evoke a response in the IC. With an increase in stimulus amplitude, the short latency neuronal response became synchronized and deterministic, with 100% firing probability for the highest amplitude of stimulation. Figure 3: Effects of pulse amplitude modulation on the IC neurons. Differential neuronal response of IC to low ( a ), intermediate ( b ) and high ( c ) amplitudes of μMS of the DCN for the same stimulation pulse-width (50 μs), while the inter-pulse interval was randomized with an average of 500 ms. The first column depicts the overlaid electrophysiological activity of the IC in response to 100 stimulation pulses delivered at each amplitude of stimulation. The second and third columns illustrate the peri-stimulus rasters and histograms of the multi-unit spiking activity, respectively. Magnetic stimulation for each plot was aligned to time equals zero. 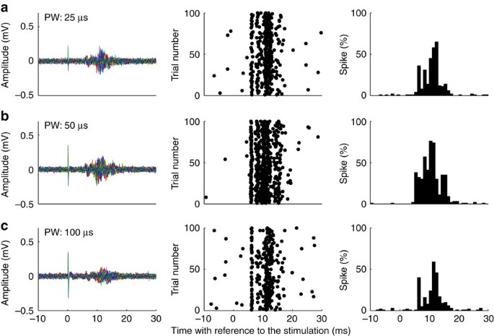Figure 4: Effects of pulse-width modulation on the IC neurons. Differential neuronal response of IC to short (a), intermediate (b) and long (c) pulse-widths of μMS of the DCN for the same stimulation pulse amplitude (300 mV), while the inter-pulse interval was randomized with the avearage of 500 ms. The first column depicts the overlaid electrophysiological activity of the IC in response to 100 stimulation pulses delivered at each pulse-width of stimulation. The second and third columns illustrate the peri-stimulus rasters and histograms of the multi-unit spiking activity, respectively. Magnetic stimulation for each plot was aligned to time equals zero. Full size image Figure 4 shows an example of the IC-evoked response for three different stimulus pulse-widths (25, 50 and 100 μs) for a single amplitude (300 mV) of stimulation in the same animal. As shown, all three pulse-widths at this amplitude resulted in activation of the IC. Interestingly, the middle pulse-width (50 μs) resulted in the greatest activation of the IC. Specifically, the average number of evoked spikes between 5 and 20 ms after stimulation with pulse-widths of 25, 50 and 100 μs were 3.1±1.2, 4.8±1.2, and 2.5±1.2 (mean±s.d. ), respectively. Statistical analysis demonstrated that the 50-μs stimulation significantly evoked more spikes compared with 25 or 100 μs ( P <0.001; Kruskal–Wallis test with Bonferroni correction, n =100 stimulus pulses per parameter). Figure 4: Effects of pulse-width modulation on the IC neurons. Differential neuronal response of IC to short ( a ), intermediate ( b ) and long ( c ) pulse-widths of μMS of the DCN for the same stimulation pulse amplitude (300 mV), while the inter-pulse interval was randomized with the avearage of 500 ms. The first column depicts the overlaid electrophysiological activity of the IC in response to 100 stimulation pulses delivered at each pulse-width of stimulation. The second and third columns illustrate the peri-stimulus rasters and histograms of the multi-unit spiking activity, respectively. Magnetic stimulation for each plot was aligned to time equals zero. Full size image Summary of IC neuronal responses to μMS of DCN In order to further evaluate the relationship between the amplitude and pulse-width of μMS, we summarized the IC-evoked potentials for all stimulation parameters tested ( Fig. 5 ). One animal was excluded from this comparison because only a single pulse-width was tested. To compare across animals, the multi-unit spike rates were normalized after each stimulus pulse (5–20 ms post stimulus onset) for each of the different parameters of stimulation. The normalization was performed by subtracting the mean baseline firing rate during the period before stimulation (−100 to −5 ms) from that during the post stimulation period. The pulse-widths were fixed at 25, 50 and 100 μs, while the amplitudes of stimulation were different for each animal, as the threshold for activation of the IC was variable between animals. Each stimulation parameter analysed consisted of 100 stimulation pulses with an average of 500 ms between two consecutive μMS pulses. As illustrated ( Fig. 5 ), the neuronal firing rate increased for all animals as the stimulation amplitude increased, regardless of pulse-width. Regarding the effects of pulse-width, in the moderate range of stimulus amplitudes (that is, above threshold but not saturated), the 50-μs pulse-width generated a stronger evoked response than either 25 μs or 100 μs pulse-widths ( P <0.001 for each animal; Kruskal–Wallis test with a Bonferroni correction, n =100 stimulus pulses per parameter). 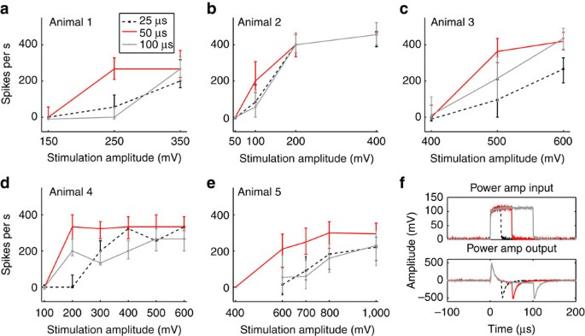Figure 5: Summary of effects of μMS amplitude and pulse-width modulation on IC activities. The spike rates between 5 ms and 20 ms after stimulation with different amplitudes and pulse-widths are displayed for each animal (n=100 stimulus pulse per stimulus parameter) (a–e). Each error bar in the figure represents the first and the third quartiles. The results indicate that the activity increased as the stimulation amplitude increased regardless of pulse-width. However, 50 μs pulse-width was more effective than 25 μs or 100 μs at certain amplitudes. Examples of the input waveforms to the power amplifier and its corresponding voltage across the coil (power amp output) are shown (f). The peak output amplitude was five times that of input amplitude. Figure 5: Summary of effects of μMS amplitude and pulse-width modulation on IC activities. The spike rates between 5 ms and 20 ms after stimulation with different amplitudes and pulse-widths are displayed for each animal ( n =100 stimulus pulse per stimulus parameter) ( a – e ). Each error bar in the figure represents the first and the third quartiles. The results indicate that the activity increased as the stimulation amplitude increased regardless of pulse-width. However, 50 μs pulse-width was more effective than 25 μs or 100 μs at certain amplitudes. Examples of the input waveforms to the power amplifier and its corresponding voltage across the coil (power amp output) are shown ( f ). The peak output amplitude was five times that of input amplitude. Full size image Control experiments In order to demonstrate that the μMS-evoked responses were biological in nature and that the neuronal responses were due to activation of the DCN, we performed two control experiments. In the first experiment, we recorded the stimulus-evoked response from the IC before and after the animal was given a lethal overdose of anaesthetic. Before the overdose was administered, a μMS stimulus that evoked a clear and robust IC response was presented ( Fig. 6a ). After overdose of anesthetics, the evoked response was completed abolished, indicating that the evoked response was biological in nature ( Fig. 6b ). 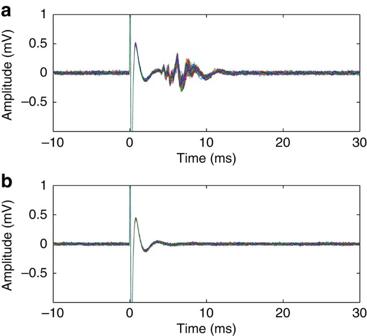Figure 6: Evoked responses of the IC due to μMS of the DCN before and after euthanasia. Neuronal responses to μMS of the DCN in the IC (a), then following euthanasia (b) in the same animal are illustrated. Each plot illustrates the overlaid electrophysiological response to 100 stimulation pulses delivered to the DCN (raw trace at same amplitude of stimulation in same animal). Figure 6: Evoked responses of the IC due to μMS of the DCN before and after euthanasia. Neuronal responses to μMS of the DCN in the IC ( a ), then following euthanasia ( b ) in the same animal are illustrated. Each plot illustrates the overlaid electrophysiological response to 100 stimulation pulses delivered to the DCN (raw trace at same amplitude of stimulation in same animal). Full size image In a second control, we sought to establish that the applied magnetic field resulted in evoked responses in the IC via direct activation of the DCN. In order to demonstrate this, we performed μMS-evoked neuronal recordings in the visual cortex, which has no known direct connections with the DCN. In addition, we recorded evoked potentials from the IC before and after the CN had been surgically ablated. As a further control, we also examined the auditory-evoked response in each recording area to demonstrate that it was present when recording from the IC and that it was absent after the CN had been ablated. The results of the second control experiments are illustrated in Fig. 7 . 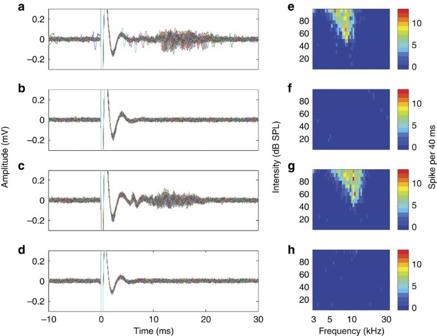Figure 7: Neuronal responses in different conditions. Neuronal response to μMS of the DCN in the IC (a), in visual cortex (b), in a second IC position (c) and then following aspiration of the CN (d) in the same animal. Each plot illustrates the overlaid electrophysiological response to 100 μMS pulses delivered to the DCN (or in the vicinity of the DCN following aspiration). The response areas (e–h) illustrate the frequency tuning of neurons at the respective recording sites for which the traces in panelsa–dwere obtained. Figure 7a,e shows the μMS- and auditory-evoked activity of the first IC recording site, respectively. As seen, the application of both μMS to the DCN and auditory stimuli resulted in robust neuronal responses in the IC. When the recording electrode was placed in the visual cortex, where there is no known direct connection from IC or CN, no μMS or auditory-evoked response could be elicited ( Fig. 7b,f ). When the recording electrode was placed back in the IC, where the μMS and auditory evoked response were originally obtained ( Fig. 7c,g ) similar to Fig. 7a,e , μMS of the DCN still reliably elicited activation of the IC, which demonstrates that the CN–IC pathway was still intact. Finally, after the CN had been ablated, the μMS- and auditory-evoked responses were abolished ( Fig. 7d,h ). The disappearance of the neuronal activities in IC evoked by sound stimulation indicates proper removal of CN and further supports that the previous μMS-evoked responses were elicited via the auditory pathway. Moreover, as the stimulus artifact waveforms were similar for all recordings, we can draw the conclusion that the activation of IC neurons was not by direct stimulation of IC, but rather via activation of pathways projecting to the IC. Figure 7: Neuronal responses in different conditions. Neuronal response to μMS of the DCN in the IC ( a ), in visual cortex ( b ), in a second IC position ( c ) and then following aspiration of the CN ( d ) in the same animal. Each plot illustrates the overlaid electrophysiological response to 100 μMS pulses delivered to the DCN (or in the vicinity of the DCN following aspiration). The response areas ( e – h ) illustrate the frequency tuning of neurons at the respective recording sites for which the traces in panels a – d were obtained. Full size image This study is the first to demonstrate that μMS is capable of activating brain circuits in the living animal. Moreover, the application of μMS did not seem to adversely alter the physiology of the animals, at least in terms of respiration, heart rate or mortality. Although we do not yet know the cellular populations activated by the applied magnetic fields, it is likely that more than one population of neurons is involved. This hypothesis is supported by the observation of two stimulation-evoked response components, including an early, synchronized response with a short latency (5–6 ms), and a later more temporally diffuse response. We propose two alternative explanations to explain the early-evoked component. The first explanation is that this activation represents direct input to the IC from the CN and possibly from the DCN itself. The early-evoked component is comparable to first spike latencies of IC neurons elicited by acoustic stimulation after correcting for processing time before the cochlear nucleus level, which were found to be in the range of 4.7–12.1 ms; they are also comparable to the first spike latencies evoked in the IC by electrical stimulation of the VCN, which ranged from 2.8 to 10.4 ms [34] . Alternatively, the early-evoked component could represent the antidromic activation of descending fibres of the IC that innervate the DCN. This postulation is supported by a number of features of the evoked response and the established anatomy of the DCN. Namely, the early-evoked component had little variation in latency regardless of the amplitude of stimulation. As antidromic responses are devoid of synaptic delays, their latencies are dependent only on the axonal conduction velocities, which are more temporally consistent and have higher transmission efficacies than trans-synaptic transmission [33] . In addition, anatomical studies of the DCN have shown that the descending fibres from the IC to the DCN innervate at the level of the fusiform cell layer [35] . As such, one would expect that as the amplitude of stimulation increased, and the magnetic fields penetrate into deeper layers of the DCN, the efficacy of eliciting the early component would increase without a concurrent change in response latency, as was consistently the case in our experiments. Although we cannot clearly ascertain the source of the early-evoked component at this time, future studies could resolve this issue by using a combination of pharmacological, transection/lesion and electrophysiological approaches. The responses of longer latency (8–20 ms) observed in the IC during μMS likely reflect the activation of other, less-direct, trans-synaptic pathways from the DCN to the IC. Indirect inputs from the DCN to the IC may include fusiform or giant cell projections to IC via the nucleus of the lateral lemniscus. Some DCN neurons (for example, tuberculoventral cells) project to the VCN, which then projects to the IC. Further spread of activation over time may result from processing delays within the IC itself that are mediated by interneurons interposed between the various pathways just mentioned and the recorded IC neurons. This multiplicity of inputs complicates the interpretation of substrates, but the specific contributions of these pathways are tractable and can be elucidated using appropriate electrophysiological and anatomical techniques. In the control experiments, we demonstrated that neuronal activation of the IC was not by direct stimulation of IC but by the activation of CN–IC pathway. The concurrent obliteration of the μMS-evoked response and frequency tuning of IC neurons after CN ablation indicate that activation of IC neurons was through CN stimulation. Moreover, if the evoked responses of the IC were due to direct activation, the latency of the responses would be much shorter than was observed. As the coil was located above the DCN surface, DCN neurons are most likely to be directly activated by the induced electric field. On the other hand, at high amplitudes of stimulation, the induced electric fields can also possibly activate the VCN, which may account for the modulation of the secondary response latencies and variance. In either case, these data demonstrate that the μMS activated IC neurons via the auditory pathway. The current study demonstrates that pulse-width of stimulation is also an important factor in governing neuronal activation with μMS. Namely, the finding that a 50-μs pulse-width evoked a greater response than either 25 or 100 μs suggests that the change in current densities induced by μMS may significantly impact the ability to generate evoked responses. As the induced electrical field intensity is proportional to the time derivative of the magnetic flux density, which is proportional to the current through the coil, we speculate that what is important is not the pulse duration but the change of current over time or the so called slew rate. This unique property would significantly distinguish μMS from electrical stimulation. Our findings are encouraging for advancing μMS as a novel neurophysiological tool. The current results, as well as prior findings, indicate that the orientation of the coils, amplitude and pulse-width of μMS can be optimized for specific experimental or therapeutic goals. Although the mechanism that governs the pulse-width effect is not fully understood, the results clearly demonstrate the need to consider the pulse-width as an important stimulation parameter for future studies. In the same way that pulse-width needs further study, the efficacy of the different magnetic stimulation waveforms needs further investigation, as is currently being explored for TMS [36] . In addition, although the effects of the brain activation states on the μMS responses were minimized by randomizing the stimulation parameters, state-dependency of μMS as demonstrated in TMS studies needs further research [25] , [37] , [38] . In closing, this study demonstrates that μMS is capable of activating a functional pathway of the brain with high degrees of temporal resolution. These findings also demonstrate that μMS can be effectively employed to explore the electrophysiological properties of brain circuits using in vivo preparations. For instance, in vivo μMS models may prove to be a valuable tool for understanding the mechanisms that underlie the therapeutic effects and optimal parameters of TMS [39] . However, before μMS can be considered as a potential therapeutic alternative to invasive electrical stimulation technologies, a number of issues need to be addressed, including safety, long-term therapeutic efficacy, energy efficiency, stimulation parameters, coil miniaturization and spatial specificity. For example, in terms of spatial specificity, the tonotopic organization of rodent DCN can be used as a tool to test the spatial selectivity of different coil designs and stimulation parameters in the future [40] . Despite these remaining challenges, this technology offers a tremendous opportunity for translational science and novel therapeutic interventions and provides several distinct advantages over traditional electrical and magnetic simulation technology. Animal subjects Adult male Syrian golden hamsters aged 12–17 weeks were acquired from Charles River Laboratory and housed in the animal vivarium of the Lerner Research Institute on a 12 hr:12 hr light:dark cycle. All procedures performed were approved by the Institutional Animal Care and Use Committee of the Cleveland Clinic, which adheres to the NIH Guide for the Care and Use of Laboratory Animals. A total of six animals were used in the current study. Surgical preparation Each animal was anaesthetised using intramuscular injection of Ketamine/Xylazine (117/18 mg kg −1 ). Animals were placed on a heating pad inside a sound-insulated booth. A rectal thermometer was inserted into the animal and its output relayed to a current regulator to keep the core temperature at 37 °C. A tracheostomy was performed using a midline neck incision. A CT-1000 cardio-tachometer (CWE Inc., Ardmore, PA, USA) was used to monitor the heart rate and the ECG waveform throughout the surgery and electrophysiological recording period. The animal was then mounted on a head brace, and an occipital and partial parietal craniectomy was performed under a Leica (MZ16F) surgical microscope. Bleeding was controlled using bone wax and gel foam until complete surgical haemostasis was achieved. A micro-aspirator was then used to remove part of the cerebellum overlying the left DCN and caudal-most part of the right cerebrum to expose the right IC. At the completion of surgery, the DCN and IC were exposed and made accessible for electrophysiological recordings. Supplements of anaesthetic were administered every 30–45 min and the heart rate was kept below 240 beats per min, indicating an adequate depth of anaesthesia during the recording session. A camera was mounted on top of a surgical microscope to view the DCN and IC from a dorsal perspective. Electrophysiological recordings Multi-unit recordings were performed in the IC using electrodes with an impedance of 0.4–0.5 MΩ [41] . The signal from the electrode was amplified (1000 × ) and bandpass-filtered (0.3–10 kHz) using a differential amplifier (DAM80, World Precision Instruments, Sarasota, FL, USA). Once conditioned, the electrophysiological data were digitized at 40 kHz (NI PCIe-6251, National Instruments, Austin, TX, USA) and archived for offline analysis. Frequency response properties were determined by counting the number of voltage events exceeding −100 μV in response to each of 800 monoaurally presented tonal stimuli (16 intensities and 50 frequencies), each lasting 30 ms (5-ms rise/fall time) and separated by an inter-stimulus interval of 50 ms [42] . The pure tones were delivered through a Beyer Dynamic DT-48 speaker coupled to the left external ear through a conical tube. The voltage events recorded were used to plot frequency response curves from which the characteristic frequency and threshold were calculated for each cluster of neurons. These measurements allowed precise localization of the recording electrode along the frequency axis of the central nucleus of the IC (CNIC). Magnetic stimulation methods In this study, in order to generate a time-varying magnetic field in the neuronal tissue, a submillimeter size non-ferromagnetic core inductor was used (see below). During the experiments, the microcoil was mounted on a second manipulator and positioned above the dorsal aspect of the DCN and could be controlled remotely from outside the recording chamber. Using the manipulator the coil was positioned ~100 μm dorsal to (not touching) the surface of the DCN. Owing to variations in the thickness of the coil insulators (~50 μm), the distance above the DCN was variable between the different coils used in the study. In order to establish activation thresholds for each animal, the output voltage of the function generator was increased in 100 mV increments (starting at 100 mV) until a clear IC post-stimulus activation could be observed. Monophasic rectangular stimulation pulses with different pulse-widths and amplitudes were generated by a function generator (AFG3012B, Tektronix Inc. Beaverton, OR, USA) triggered by an analogue I/O card (NI PCIe-6251, National Instruments), with an average rate of 2 Hz. The pulses were then amplified by a 1,000-W audio amplifier (PB717X, Pyramid Inc., Brooklyn, NY, USA) and applied to the microcoil for magnetic field generation. The input pulse to the power amplifier and the corresponding output waveform of the power amplifier are shown in Fig. 5f . The outputs of both the power amplifier and the generator were connected to BNC splitters for monitoring with an oscilloscope (DPO3012, Tektronix Inc., Beaverton, OR, USA). When referencing ‘stimulus amplitude’ in this paper, we indicate only the input pulse amplitude to the power amplifier. In order to prevent the carrying over effect from the previous trial, the order of the stimulation parameters (pulse amplitude and pulse-width) was randomized for each animal in addition to allowing 30 s resting periods between each 60 s. Construction of coils A commercial multilayer MEMS RF 0402 inductor (ELJ-RFR10JFB, Panasonic Electronic Devices Corporation of America (PEDCA), Knoxville, TN, USA) with square helical shape, 21 turns, 100 nH inductance, 5.5 Ω maximum DC resistance, Q (100 MHz) of 8, self-resonant or maximum frequency of 1.25 GHz, and 400 × 400 × 600 μm size (uninsulated dimension) was soldered using a 15-mils 44-resin core solder SN63PB37 (Kester, Itasca, IL, USA) on the tip of 34-AWG copper wires with polyimide enamel inner coat and polyurethane over coat (Philmore Mfg., Rockford, IL, USA). The two wires were then inserted in a 16¾ G blunt cannula with 150 mm of length. The needle was inserted in a 1-ml syringe and two electrical wires inside were connected to a BNC connector. The BNC was glued with a hot-melt adhesive to the syringe, which was then secured to the micromanipulator during the experiments. Finally, the μMS coils were coated with acrylatecopolymer enamel (Revlon, New York, NY, USA) for electrical insulation and water impermeability of the exposed coil terminals. The μMS coils were thoroughly tested to make sure that the current leak would remain minimal during the magnetic stimulation experiments. This test was important because, if present, such currents could have produced the observed neural stimulation. The test consisted of measuring the insulators impedance by submersing the coils in a physiological solution (0.9% NaCl) together with an electrode. The impedance between each terminal of the μMS coil and the electrode in the solution was measured with a commercial impedance meter (Omega-Tip-Z, World Precision Instruments) immediately before and after each experiment. The coils were considered well insulated only when this impedance was >2 MΩ. In addition, the resistance across the microcoil was also tested before and after each experiment using a multimeter (Fluke 115 Digital Multimeter, Everett, WA, USA), with normal values ranging from 4.5 to 4.7 Ω. The magnetic flux density and the induced electric field intensity using the same coil have been previously demonstrated in computer simulation using a finite element method software COMSOL Multiphysics 4.2a with the AC/DC module (COMSOL, Burlington, MA, USA) [32] . Analysis of stimulation data A multi-unit analysis method was used to detect the neuronal activities in IC. For this analysis, the stimulus artifact in the IC recording was removed or attenuated using a curve fitting method [43] . In this method, the stimulus artifact waveform was considered to be the result of linear LCR circuits. Therefore, the artifact waveform was assumed to be the multiplication of the exponential decay term and sinusoidal term as a result of linear system. In the curve fitting method, the parameters were found minimizing the following cost function L in the following equations. where x S ( t ) is the stimulus artifact, and a , b , c and d are the parameters to be estimated. In this equation, t 1 =1 ms, t 2 =5 ms, t 3 =10 ms and t 4 =30 ms were selected so that x S ( t ) follows the recorded stimulus artifact waveform between t 1 and t 2 and decays to zero after t 3 . For the curve fitting function, the least squares error method (that is, lsqrcurvefit) was used in MATLAB (The MathWorks Inc., Natick, MA, USA). After the curve fitting, the artifact was subtracted from the recorded waveform, while the time period from 0–1 ms after the stimulation was set to zero. Once the stimulus artifact was reduced, multi-unit spike units were detected using Offline Sorter (Plexon Inc, Dallas, TX, USA). Statistical analysis Statistical analyses were applied to the multi-unit data ( n =100) in order to determine differences between μ MS parameters (pulse-width and amplitudes). Statistical significance was accepted with P <0.001 using a Kruskal–Wallis test with a Bonferroni correction for multiple comparisons. How to cite this article: Park, H. -J. et al. Activation of the central nervous system induced by micro-magnetic stimulation. Nat. Commun. 4:2463 doi: 10.1038/ncomms3463 (2013).